A recoverable state of axon injury persists for hours after spinal cord contusionin vivo Therapeutic strategies for spinal cord injury (SCI) commonly focus on regenerating disconnected axons. An alternative approach would be to maintain continuity of damaged axons, especially after contusion. The viability of such neuropreservative strategies depends on the degree to which initially injured axons can recover. Here we use morphological and molecular in vivo imaging after contusion SCI in mice to show that injured axons persist in a metastable state for hours. Intra-axonal calcium dynamics influence fate, but the outcome is not invariably destructive in that many axons with calcium elevations recover homeostasis without intervention. Calcium enters axons primarily through mechanopores. Spontaneous pore resealing allows calcium levels to normalize and axons to survive long term. Axon loss can be halted by blocking calcium influx or calpain, even with delayed initiation. Our data identify an inherent self-preservation process in contused axons and a window of opportunity for rescuing connectivity after nontransecting SCI. The extent of axon damage is an important predictor of clinical outcome following a multitude of central nervous system pathologies including those caused by ischaemia, inflammation and trauma [1] , [2] . For spinal cord injury (SCI) in particular, where communication between the brain and sites distal to the lesion depends on projecting axons in white matter tracts, the number of axons that survive the injury makes a significant difference in behavioural parameters of experimental models [3] , [4] and quality of life for human patients [5] . The quest for therapeutic options to improve the outcome of SCI so far has mainly focused on neuronal repair or replacement [6] . Such neurorestorative approaches could substantially benefit from increasing preservation of still connected axons, with such spared axons serving as guide structures for re-growth, as synaptic partners or trophic targets for transplanted cells and as substrates for remodelling and plasticity. Thus, optimally any neurorestorative therapy would be preceded by an acute neuropreservative intervention, as for example successfully employed in stroke, where re-establishing perfusion in time allows rescuing hypoxic neurons [7] . Therefore, whether axons can actually recover from an initial trauma, which mechanisms determine survival and how recovery could be promoted are important questions in devising a comprehensive treatment strategy aimed at preserving and restoring spinal function. For obvious reasons, determining spontaneous survival rates is challenging with conventional static tools of analysis that capture the morphological state of spinal axons once at a single time point and depend on inferring the original degree of damage from the lesion size or other surrogate measures [8] . Especially in the clinically relevant contusion injury models, such inferences are difficult, as no simple marker for previous injury exists. In contrast, in vivo imaging of the structural and functional state of spinal axons would provide a direct read-out of the degree of initial injury, as well as of spontaneous and therapy-induced recovery [9] . Here we have pursued this approach in the dorsal spinal cord of mice after standardized contusion injury to ask: (i) whether spontaneously recovering axons exist; (ii) which factors determine an axon’s fate; and (iii) whether axons that would have normally degenerated can be rescued during the acute injury phase. Our results demonstrate that many axons after a contusion enter a metastable state of elevated calcium and swelling, which persists for several hours and can spontaneously progress to overt fragmentation or revert to normal. We find that mechanically induced pores underlie the initial calcium influx. Failure to reseal such mechanopores over the first hours after injury predicts axonal demise. Still, the deleterious effects of intra-axonal calcium can be halted by blocking downstream pathways, and axons that survive the initial risk period maintain connectivity over long periods of time. Recovery and loss of axons occurs for several hours after contusion To follow the evolution of axonal damage in vivo in a clinically relevant model of SCI, we induced standardized spinal contusion lesions [10] in transgenic mice ( Thy1 -YFP16 (ref. 11 ); for line information, see Methods), which express yellow fluorescent protein (YFP) in many spinal axons. We impacted the dorsal surface of the exposed lumbar spinal segments (L) 4/5 with a force of 29–43 kDynes to produce superficial contusion lesions without extensive superficial bleeding or cord deformation. In vivo multiphoton microscopy within the lesion epicentre ( Fig. 1a ) allowed us to track axonal morphology and fate over the first hours after contusion. We observed a range of injury-induced axon morphologies, including apparently unaffected, swollen and broken axons (either end bulbs or fragment trails; Fig. 1b ). Time-lapse recordings revealed that, while all broken axons first swelled, swollen axons could also spontaneously recover ( Fig. 1c ; Supplementary Movie 1 ). To obtain a more quantitative view of axonal changes, we tracked the individual fate of nearly 200 axons for 240 min post injury (p.i. ; Fig. 1d ). Our results show that most swellings appeared within the first 30 min after contusion and could be stable for extended periods of time, with 38.6±6.5% (mean±s.e.m. ; n =4 mice) of swollen axons persisting beyond the 4-h observation period. This indicates that a time window exists, during which swollen axons can either proceed to fragmentation or recover. Indeed, we observed morphological recoveries of swollen axons with a similar frequency as axonal breakdowns during the first 4 h p.i. (0.122±0.042 sustained recoveries per swollen axon h versus 0.161±0.081 breakdowns per swollen axon h; mean±s.e.m. ; n =4 mice). Notably, fragmentation and recovery rates were rather stable over the entire observation period, indicating that the critical window for axonal fate decisions likely extends even beyond our 4-h observation period (0.127±0.060 versus 0.092±0.037 for recoveries and 0.152±0.083 versus 0.177±0.082 for breakdowns in the first 2 versus last 2 h p.i. ; mean±s.e.m. ; n =4 mice). 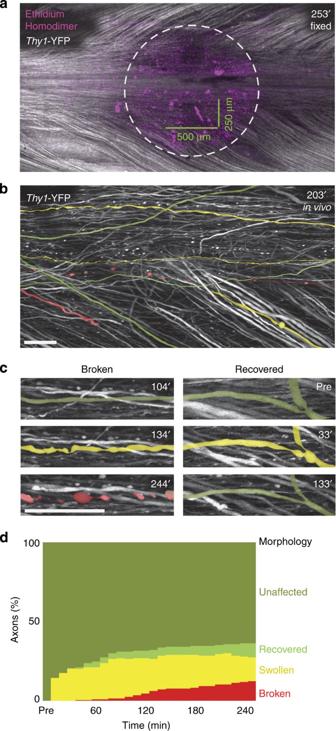Figure 1: Axons that swell following spinal contusion can break down or recover. (a) Low-magnification confocal image showing the extent of damage 4-h p.i. in a fixed spinal cord whole-mount derived from a transgenicThy1-YFP16 mouse (greyscale). Dying cells were labelled by incubation with ethidium homodimer (magenta) revealing the location of the contusion area (dashed circle). The approximate dimensions of the field of view obtained fromin vivotime-lapse montages are shown by green scale bars. (b) Single frame (montaged maximum intensity projection) from a multiphotonin vivotime-lapse showing the range of axonal morphologies present after contusion including healthy appearing (pseudocoloured green), swollen (yellow) and broken (red). (c) Magnified details fromin vivotime-lapse recordings showing typical changes in axonal morphology at the indicated times as min p.i. (‘pre’: before injury). Swollen axons can progress to a broken state (left panel); however, spontaneous recovery events are also observed (right panel; axons pseudocoloured as inb;Thy1-YFP16 line). (d) Graph showing the morphological changes of a large population of contused axons (194 axons, 4Thy1-YFP16 mice). Scale bars inb,c, 20 μm. Figure 1: Axons that swell following spinal contusion can break down or recover. ( a ) Low-magnification confocal image showing the extent of damage 4-h p.i. in a fixed spinal cord whole-mount derived from a transgenic Thy1 -YFP16 mouse (greyscale). Dying cells were labelled by incubation with ethidium homodimer (magenta) revealing the location of the contusion area (dashed circle). The approximate dimensions of the field of view obtained from in vivo time-lapse montages are shown by green scale bars. ( b ) Single frame (montaged maximum intensity projection) from a multiphoton in vivo time-lapse showing the range of axonal morphologies present after contusion including healthy appearing (pseudocoloured green), swollen (yellow) and broken (red). ( c ) Magnified details from in vivo time-lapse recordings showing typical changes in axonal morphology at the indicated times as min p.i. (‘pre’: before injury). Swollen axons can progress to a broken state (left panel); however, spontaneous recovery events are also observed (right panel; axons pseudocoloured as in b ; Thy1 -YFP16 line). ( d ) Graph showing the morphological changes of a large population of contused axons (194 axons, 4 Thy1 -YFP16 mice). Scale bars in b , c , 20 μm. Full size image Calcium dynamics predict axonal fate after contusion While increased calcium levels in other neurological conditions have been generally considered to signal the imminent demise of neurons and axons [2] , [12] , we wondered how calcium dynamics relate to the balance of axonal loss and recovery in the contusion model. Thus, we examined the calcium handling of axons using Thy1 -TNXXL transgenic mice, which neuronally express a fluorescence resonance energy transfer (FRET)-based calcium sensor [13] ( Fig. 2a ; Supplementary Movie 2 ), and label axon populations with a distinct but overlapping caliber distribution compared with the Thy -YFP16 transgenic line ( Supplementary Fig. 1 ). We found that over half of the axons showed elevated intra-axonal calcium levels at the first observation time point after injury (2–8 min; for details see Methods). Over time, elevated calcium levels recovered to normal in some axons, while they persisted in others, which often later fragmented ( Fig. 2b,c ). 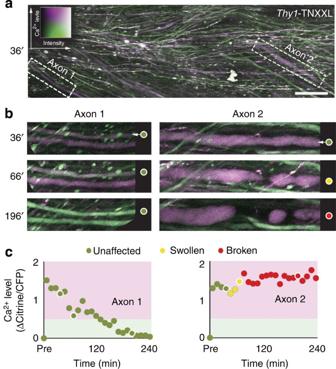Figure 2: Calcium elevations can spontaneously recover or lead to axonal breakdown. (a) Single time point (montaged maximum intensity projection) from a multiphotonin vivotime-lapse showing axonal calcium levels app. half an hour p.i. (Thy1-TNXXL line; see colour look-up table in left corner). (b) Example frames (areas boxed ina) showing an axon that returns to normal intra-axonal Ca2+levels without morphological change (Axon 1, left) and an axon that fragments without return to normal Ca2+levels (Axon 2, right). Indicated time points are p.i.; coloured circles indicate morphological state of the axons tracked inc. (c) Changes in FRET ratios (Δ Citrine/CFP) from pre-injury baseline (‘pre’) for the axons shown inb. Circled data points indicate time points shown inb. The cutoff between calcium-normal and -elevated axons (δCitrine/CFP=+0.5) is colour-coded(green and magenta, respectively). Scale bar ina, 20 μm. Figure 2: Calcium elevations can spontaneously recover or lead to axonal breakdown. ( a ) Single time point (montaged maximum intensity projection) from a multiphoton in vivo time-lapse showing axonal calcium levels app. half an hour p.i. ( Thy1 -TNXXL line; see colour look-up table in left corner). ( b ) Example frames (areas boxed in a ) showing an axon that returns to normal intra-axonal Ca 2+ levels without morphological change (Axon 1, left) and an axon that fragments without return to normal Ca 2+ levels (Axon 2, right). Indicated time points are p.i. ; coloured circles indicate morphological state of the axons tracked in c . ( c ) Changes in FRET ratios (Δ Citrine/CFP) from pre-injury baseline (‘pre’) for the axons shown in b . Circled data points indicate time points shown in b . The cutoff between calcium-normal and -elevated axons (δCitrine/CFP=+0.5) is colour-coded(green and magenta, respectively). Scale bar in a , 20 μm. Full size image On a population level, the pattern of axonal swelling followed by recovery or breakdown was similar to that seen for Thy1 -YFP16 ( Fig. 3a , Supplementary Fig. 1 ). Most calcium recoveries occurred within 100 min p.i. (70.4±5.5%; mean±s.e.m. ; n =10 mice). After 100 min, recovery slowed (calcium recovery rate: 0.507±0.074 calcium recoveries per axon h from 0 to 100 min p.i. versus 0.293±0.068 from 100 to 240 min p.i. ; mean±s.e.m. ; n =10 mice) and increased calcium levels persisted in many axons ( Fig. 3b ). To determine the predictive value of calcium dynamics, we inquired how previous calcium history influenced axonal survival. Axonal fragmentation was almost exclusively observed in axons with an initial calcium rise (0.081±0.014 breakdowns per axon h for calcium-elevated axons versus 0.005±0.003 for calcium normal; mean±s.e.m. ; n =10 mice; Fig. 3c ). Still, a sizeable fraction of calcium-normal axons initially swelled. This seemed to be mostly the case for thinner axons, while propensity for initial calcium rise and fragmentation was largely independent of calibre ( Supplementary Fig. 2a,b ). Interestingly, our data also revealed that axons with an initial calcium rise could still ensure their survival by delayed calcium clearance. Axons that returned to normal calcium levels during the initial recovery phase (≤100 min p.i.) were largely protected from fragmentation (0.016±0.010 breakdowns per axon h; mean±s.e.m. ; n =10 mice) compared with those axons in which elevated calcium levels persisted (0.160±0.037; mean±s.e.m. ; n =10 mice; P <0.001 Mann–Whitney U -test; Fig. 3d ). 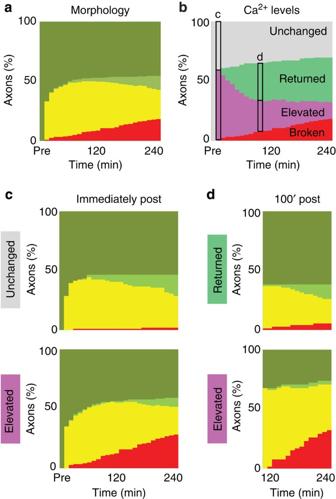Figure 3: Calcium handling of contused axons predicts their fate. Population data of morphological (a) and Ca2+changes (b) in contused axons (248 axons, 10Thy1-TNXXL mice). Axons with initially normal Ca2+levels were compared with those with immediate elevations after contusion (c, top and bottom, respectively). Similarly, axons were divided into those which had returned Ca2+levels to normal by 100 min or those that had not (d, top and bottom, respectively). Figure 3: Calcium handling of contused axons predicts their fate. Population data of morphological ( a ) and Ca 2+ changes ( b ) in contused axons (248 axons, 10 Thy1 -TNXXL mice). Axons with initially normal Ca 2+ levels were compared with those with immediate elevations after contusion ( c , top and bottom, respectively). Similarly, axons were divided into those which had returned Ca 2+ levels to normal by 100 min or those that had not ( d , top and bottom, respectively). Full size image While calcium elevations predicted axonal fate, it is possible that calcium is simply correlated to injury severity, but not a driving force of degeneration. To directly assess this, we removed extracellular calcium for the first hour after injury and re-introduced calcium for the remaining 3 h ( Fig. 4 ; Supplementary Movie 3 ). EGTA treatment was effective in preventing sustained calcium elevations and resolved 76.2±7.5% (mean±s.e.m. ; n =6 mice) of those that had already occurred. During the calcium removal period, no axons fragmented. However, after calcium was re-introduced and axonal calcium levels rose, breakdown began within an hour at an accelerated rate ( Fig. 4b ). In line with our previous results, some axonal swellings (mostly in thin axons; Supplementary Fig. 2c ) were still apparent in the absence of calcium. Taken together, calcium handling over the first hours after injury critically determines whether an axon survives or succumbs. Notably, we observed that not only those axons that lack an initial calcium elevation but also those that managed to correct the initial calcium rise are protected from fragmentation—opening a window for interventions to clear calcium or inhibit downstream degeneration pathways. 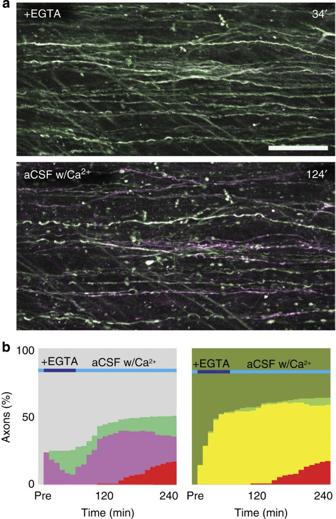Figure 4: Removal of extracellular Ca2+blocks axonal fragmentationin vivo. (a) Single time points (montaged maximum intensity projection) from a multiphotonin vivotime-lapse showing axonal calcium levels after contusion in the absence of extracellular Ca2+(top; ‘+EGTA’: 0 Ca2+aCSF containing 25 mM EGTA—these high levels were required because of restrictedin vivoaccess) and after return to normal Ca2+(bottom; ‘aCSF w/Ca2+’). For colour look-up tablecf.Fig. 2a. (b) Population data of Ca2+(left) and morphological changes (right) from such experiments (170 axons, 6Thy1-TNXXL mice; for a comparable control,cf.Fig. 5c,e). Scale bar ina, 20 μm. Figure 4: Removal of extracellular Ca 2+ blocks axonal fragmentation in vivo . ( a ) Single time points (montaged maximum intensity projection) from a multiphoton in vivo time-lapse showing axonal calcium levels after contusion in the absence of extracellular Ca 2+ (top; ‘+EGTA’: 0 Ca 2+ aCSF containing 25 mM EGTA—these high levels were required because of restricted in vivo access) and after return to normal Ca 2+ (bottom; ‘aCSF w/Ca 2+ ’). For colour look-up table cf. Fig. 2a . ( b ) Population data of Ca 2+ (left) and morphological changes (right) from such experiments (170 axons, 6 Thy1 -TNXXL mice; for a comparable control, cf. Fig. 5c,e ). Scale bar in a , 20 μm. Full size image At-risk axons can be rescued in the first hours post injury To determine whether axons that are at risk of fragmentation can still be rescued by therapeutic interventions initiated after injury, we pharmacologically inhibited the activity of calpain, a calcium-dependent protease implicated in axonal fragmentation [14] , [15] , [16] . We applied calpain inhibitor III during the second hour p.i., which protected axons out to 4 h p.i. (calpain inhibitor: 0.005±0.002 breakdowns per axon h versus vehicle: 0.048±0.011; mean±s.e.m. ; n =6 and 7 mice, respectively; P <0.01 Mann–Whitney U -test; Fig. 5a,b ). To examine whether calpain inhibition would continue to protect axons, we extended our observation window to 8 h p.i. Although only including samples that survived to 8 h after injury seemed to bias for weaker lesions, there was a reduction in axonal breakdown in calpain inhibitor-treated mice versus dimethylsulphoxide (DMSO) control treatment (calpain inhibitor: 0.005±0.002 breakdowns per axon h versus vehicle: 0.016±0.004; mean±s.e.m. ; n =5 and 4 mice, respectively; P =0.05 Mann–Whitney U -test; Fig. 5c–f ). Calpain inhibition even rescued axons that had elevated calcium at 100 min and were hence normally at high risk of fragmentation (calpain inhibitor: 0.012±0.008 breakdowns per axon h versus vehicle: 0.081±0.017; mean±s.e.m. ; n =5 and 4 mice, respectively; P <0.05 Mann–Whitney U -test; Fig. 5g,h ). 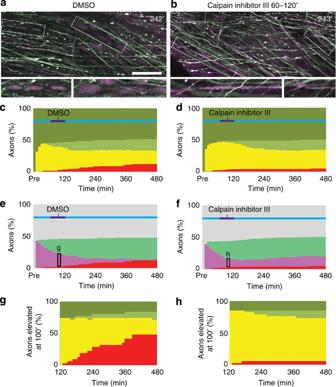Figure 5: Damaged axons can be rescued by delayed calpain inhibition. (a) Maximum intensity projection montages from a control experiment (dimethyl sulfoxide, DMSO application) and an experiment with calpain inhibitor III application (b) from 1 to 2-h p.i. Under control conditions, many calcium-elevated (magenta) axons have fragmented, while they are protected by calpain inhibition. Note that insets inahave been adjusted to more clearly show dim axonal fragments. For colour look-up tablecf.Fig. 2a. (c,d) Calpain inhibitor-treated axons swell, but do not fragment for up to 8 h after contusion, even though intra-axonal calcium levels remain elevated (e,f; DMSO: 164 axons, 4 mice, versus calpain inhibitor III: 270 axons, 5 mice). (g,h) Calpain inhibition also protects at-risk axons (that is, those that have elevated calcium at 100-min p.i.; population boxed ine,f). Scale bar ina,b, 20 μm. Figure 5: Damaged axons can be rescued by delayed calpain inhibition. ( a ) Maximum intensity projection montages from a control experiment (dimethyl sulfoxide, DMSO application) and an experiment with calpain inhibitor III application ( b ) from 1 to 2-h p.i. Under control conditions, many calcium-elevated (magenta) axons have fragmented, while they are protected by calpain inhibition. Note that insets in a have been adjusted to more clearly show dim axonal fragments. For colour look-up table cf. Fig. 2a . ( c , d ) Calpain inhibitor-treated axons swell, but do not fragment for up to 8 h after contusion, even though intra-axonal calcium levels remain elevated ( e , f ; DMSO: 164 axons, 4 mice, versus calpain inhibitor III: 270 axons, 5 mice). ( g , h ) Calpain inhibition also protects at-risk axons (that is, those that have elevated calcium at 100-min p.i. ; population boxed in e , f ). Scale bar in a , b , 20 μm. Full size image Calcium entering via mechanopores drives axonal breakdown We next sought to determine the source of elevated calcium in contused axons. The immediate rise in calcium after injury and our EGTA experiments suggested an extracellular source of calcium. Therefore, we performed a series of pilot experiments that pharmacologically queried established molecularly defined entry pathways (for example, voltage-gated calcium channels [17] , [18] , [19] ; reverse action of the sodium–calcium exchanger [20] , [21] , [22] ; glutamate receptors [23] ). These experiments failed to show strong effects on initial calcium rises (proportion of calcium-elevated axons at initial p.i. time point compared with vehicle-treated controls: 0.99±0.14, 0.98±0.11 and 1.06±0.01-fold; mean±s.e.m. ; for treatments blocking voltage-gated calcium channels, three mice, 140 axons; the Na + /Ca 2+ exchanger, three mice, 116 axons; and glutamate receptors, three mice, 111 axons, respectively) or cumulative breakdown rates (relative rate: 1.23±0.09; 1.26±0.08; and 1.26±0.22-fold; mean±s.e.m. ; compared with controls for treatments blocking voltage-gated calcium channels, the Na + /Ca 2+ exchanger and glutamate receptors, respectively, for more details see Methods). We then investigated the formation of mechanopores (holes in the plasma membrane induced by mechanical strain) as have been previously observed after central nervous system trauma [24] , [25] . Before contusion, we subdurally loaded fluorescently conjugated macromolecules (0.8 kD cadaverine or 10 kD dextran), which were excluded from axons in the healthy spinal cord ( Fig. 6a ). After contusion, however, a number of axons took up these dyes throughout their cytoplasm, indicating the presence of membrane disruptions ( Fig. 6a,b ). Cadaverine conjugates labelled more calcium-elevated axons (76±3% of axons; mean±s.e.m. ; n =3 mice) than 10 kD dextrans (62±11%; mean±s.e.m. ; n =5 mice), suggesting the presence of a range of pore sizes. We next performed a time series of cadaverine-loading experiments to explore whether dye uptake matched with sustained calcium elevations that prime later degeneration ( Fig. 6b–e ). Immediately after the contusion, the vast majority of calcium-elevated axons, but also about half of the axons with apparently normal calcium levels, took up the cadaverine dye. This suggests that some short-lasting membrane disruptions existed, which resolved before our first calcium recording. In contrast, when we performed dye-loading at 15 min p.i., the majority of dye-labelled (and thus likely porated) axons showed elevated calcium levels, while only few dye-negative axons did ( Fig. 6b,c ). Dye uptake decreased over time in calcium-elevated axons; however, a substantial fraction of calcium-elevated axons still had pores at 60 min p.i., which largely resolved 1 h later ( Fig. 6e ). 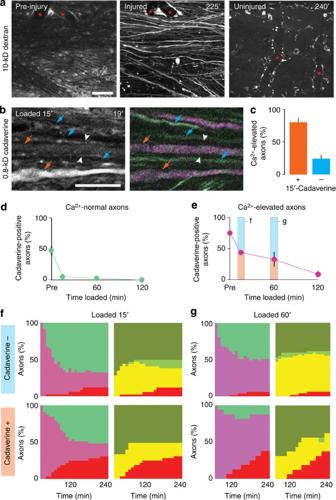Figure 6: Mechanoporation is the primary source of intra-axonal calcium after contusion. (a) Subdurally loaded dye (10 kD dextran) was excluded from uninjured axons, which were revealed by ‘negative’ staining (left, maximum intensity projection of 20 optical planes). After contusion, a number of axons took up the dye (centre, same sample as left, maximum intensity projection). Without injury, labelling is cleared from extracellular space and becomes restricted to blood vessels (asterisks) and some superficial cells (right, maximum intensity projection). Images are individually adjusted to best reveal patterns of dye distribution. (b) Axonal dye uptake after delayed loading (0.8 kD cadaverine) correlated with elevations in axonal Ca2+level (dye-positive axons, orange arrows; dye-negative axons, cyan arrows; white arrowheads indicate presumptive myelin sheaths that are also dye-positive; single optical plane from anin vivotime-lapse experiment). For colour look-up tablecf.Fig. 2a. (c) Percentage of Ca2+-elevated axons that are cadaverine-positive or -negative at the first time point (19–22-min p.i.) following dye-loading at 15-min p.i. (202 axons, 3Thy1-TNXXL mice). (d,e) Time course of dye uptake (0.8-kD cadaverine) in axons with normal Ca2+levels (d, 565 axons, 15Thy1-TNXXL mice) and in Ca2+-elevated axons (e, 226 axons, 15Thy1-TNXXL mice). (f) Ca2+(left) and morphological (right) changes in axons with elevated Ca2+at 15-min p.i., subdivided into the dye-negative (top; 34 axons, 3 mice) and -positive (lower; 33 axons, 3 mice) axon populations. (g) Ca2+(left) and morphological (right) changes in axons with elevated Ca2+at 60-min p.i., subdivided into the dye-negative (top; 47 axons, 5 mice) and -positive (lower; 16 axons, 5 mice) axon populations. Scale bars ina,b, 20 μm. Note that ind,csome error bars are hidden behind data symbols. Figure 6: Mechanoporation is the primary source of intra-axonal calcium after contusion. ( a ) Subdurally loaded dye (10 kD dextran) was excluded from uninjured axons, which were revealed by ‘negative’ staining (left, maximum intensity projection of 20 optical planes). After contusion, a number of axons took up the dye (centre, same sample as left, maximum intensity projection). Without injury, labelling is cleared from extracellular space and becomes restricted to blood vessels (asterisks) and some superficial cells (right, maximum intensity projection). Images are individually adjusted to best reveal patterns of dye distribution. ( b ) Axonal dye uptake after delayed loading (0.8 kD cadaverine) correlated with elevations in axonal Ca 2+ level (dye-positive axons, orange arrows; dye-negative axons, cyan arrows; white arrowheads indicate presumptive myelin sheaths that are also dye-positive; single optical plane from an in vivo time-lapse experiment). For colour look-up table cf. Fig. 2a . ( c ) Percentage of Ca 2+ -elevated axons that are cadaverine-positive or -negative at the first time point (19–22-min p.i.) following dye-loading at 15-min p.i. (202 axons, 3 Thy1 -TNXXL mice). ( d , e ) Time course of dye uptake (0.8-kD cadaverine) in axons with normal Ca 2+ levels ( d , 565 axons, 15 Thy1 -TNXXL mice) and in Ca 2+ -elevated axons ( e , 226 axons, 15 Thy1 -TNXXL mice). ( f ) Ca 2+ (left) and morphological (right) changes in axons with elevated Ca 2+ at 15-min p.i., subdivided into the dye-negative (top; 34 axons, 3 mice) and -positive (lower; 33 axons, 3 mice) axon populations. ( g ) Ca 2+ (left) and morphological (right) changes in axons with elevated Ca 2+ at 60-min p.i., subdivided into the dye-negative (top; 47 axons, 5 mice) and -positive (lower; 16 axons, 5 mice) axon populations. Scale bars in a , b , 20 μm. Note that in d , c some error bars are hidden behind data symbols. Full size image To assess whether the failure or success of this resealing process explains the divergent fate of axons, we determined whether calcium-elevated axons at 15 and 60 min p.i. were at higher risk if they still showed dye uptake. Axons that had been successfully resealed by 15 min (and hence did not take up dye at 15 min p.i.) tended to return to normal calcium levels slightly more often ( Fig. 6f ) and with less fragmentation (dye-positive: 0.066±.022 breakdowns per axon h versus dye-negative: 0.033±.006; mean±s.e.m. ; n =3 mice; P =0.13 Mann–Whitney U -test). Similarly, axons that successfully resealed in the first hour returned to normal calcium levels more rapidly and more often than axons that failed to reseal ( Fig. 6g ). The decreased rate of calcium recovery in the 60-min group is likely due to a confluence of axonal breakdown from the high-calcium pool, and a delay in mechanopore resealing and subsequent return to calcium homeostasis for surviving axons. Furthermore, although both populations showed a similar frequency of swellings, axonal fragmentation was significantly more likely in axons that failed to reseal (dye-positive: 0.232±.072 breakdowns per axon h versus dye-negative: 0.019±.008; mean±s.e.m. ; n =5 mice; P <0.05 Mann–Whitney U -test; Fig. 6g ). Thus, not only are mechanopores likely responsible for the majority of calcium elevations, their resolution is also protective against further calcium exposure and eventual axonal fragmentation. Axons that recover from the contusion can survive long term Finally we wanted to determine whether axons that resealed in time to recover would be able to survive long term, and thereby help to preserve neurological function. Here we took advantage of the fact that dextrans taken up via mechanopores can also serve as injury-specific tracers. We combined this with conventional anterograde and retrograde tracing to determine the fate of initially porated axons. Indeed 1 week p.i., neuronal somata labelled with a 3-kD dextran, which was loaded at the contusion site before injury, were present in adjacent dorsal root ganglia (DRGs) with almost no labelling in uninjured animals (injured: 166.5±50.2 versus uninjured: 1.3±0.6 labelled somata/DRG; mean±s.e.m. ; 10 DRGs, 5 mice per condition; Fig. 7a,b ). To demonstrate that such neurons maintained lesion-spanning projections to the thoracic spinal cord, we loaded a differently conjugated 3 kD dextran via a midthoracic dorsolateral hemisection 1 day after injury. As expected, we observed a contusion-related drop in the number of somata labelled by such delayed tracing (for details see Methods). However, a substantial fraction of such somata showed the contusion-related label (27±4%; mean±s.e.m. ; n =5 mice; Fig. 7b ) at 7 days p.i., indicating that they maintained lesion-spanning axons that were initially porated. 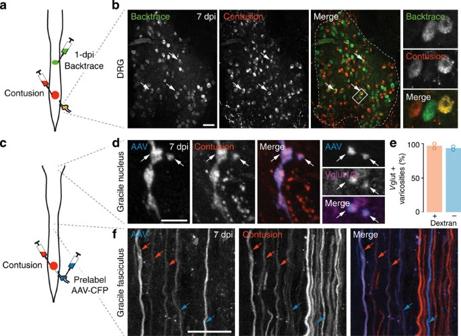Figure 7: Recovered axons can survive long term and maintain presynaptic boutons after spinal contusion. (a) Schematic representation of retrograde tracing experiments. Contusions were performed in the presence of dextran (3 kD, orange; ‘Contusion’) to retrogradely label somata in DRGs caudal to the contusion. One day p.i. axons were backtraced from the midthoracic spinal cord with differentially conjugated dextran (3 kD, green; ‘Backtrace’); 1 week p.i. caudal DRGs were collected for analysis. (b) Co-labelling of somata with both dyes was evident (arrows; maximum intensity projections of whole-mount DRGs, outlined by dashed line in ‘Merge’). Right inset is indicated by white box in ‘Merge’. (c) Schematic representation of anterograde tracing experiments. One week before contusion, an AAV driving CFP expression (blue; ‘AAV’) was injected into the L5 or L6 DRG. Lesions were performed rostrally in the presence of dextran (10 kD, orange; ‘Contusion’), and tissue was collected 1 week injury p.i. (d) AAV-labelled axon terminals (left and blue in ‘Merge’) in the gracile nucleus, which have survived the contusion, as they are also labelled with a dye (centre; orange; rotated 3D renderings). The inset shows that the varicosities (arrows) on this projection could be immunolabelled with the presynaptic marker Vglut1/2 (magenta in inset; maximum intensity projection of two optical planes spaced by 0.5 μm). (e) Quantification of Vglut1/2 staining in dextran-negative and -positive axons (186 varicosities, 2 mice). (f) Numerous AAV-positive axons (left, blue) persist in the thoracic spinal cord and also contain dye-labelling (10 kD dextran; centre, orange; maximum intensity projections with dye-positive axons indicated with orange arrows, and dye-negative axons with blue arrows, degree of dye-labelling was individually confirmed for each axon in single planes). Scale bar inb, 100 μm; ind, 5 μm and inf, 20 μm. Figure 7: Recovered axons can survive long term and maintain presynaptic boutons after spinal contusion. ( a ) Schematic representation of retrograde tracing experiments. Contusions were performed in the presence of dextran (3 kD, orange; ‘Contusion’) to retrogradely label somata in DRGs caudal to the contusion. One day p.i. axons were backtraced from the midthoracic spinal cord with differentially conjugated dextran (3 kD, green; ‘Backtrace’); 1 week p.i. caudal DRGs were collected for analysis. ( b ) Co-labelling of somata with both dyes was evident (arrows; maximum intensity projections of whole-mount DRGs, outlined by dashed line in ‘Merge’). Right inset is indicated by white box in ‘Merge’. ( c ) Schematic representation of anterograde tracing experiments. One week before contusion, an AAV driving CFP expression (blue; ‘AAV’) was injected into the L5 or L6 DRG. Lesions were performed rostrally in the presence of dextran (10 kD, orange; ‘Contusion’), and tissue was collected 1 week injury p.i. ( d ) AAV-labelled axon terminals (left and blue in ‘Merge’) in the gracile nucleus, which have survived the contusion, as they are also labelled with a dye (centre; orange; rotated 3D renderings). The inset shows that the varicosities (arrows) on this projection could be immunolabelled with the presynaptic marker Vglut1/2 (magenta in inset; maximum intensity projection of two optical planes spaced by 0.5 μm). ( e ) Quantification of Vglut1/2 staining in dextran-negative and -positive axons (186 varicosities, 2 mice). ( f ) Numerous AAV-positive axons (left, blue) persist in the thoracic spinal cord and also contain dye-labelling (10 kD dextran; centre, orange; maximum intensity projections with dye-positive axons indicated with orange arrows, and dye-negative axons with blue arrows, degree of dye-labelling was individually confirmed for each axon in single planes). Scale bar in b , 100 μm; in d , 5 μm and in f , 20 μm. Full size image To also investigate whether such recovered axons maintained long-distance connectivity, we anterogradely traced DRG axons, which originated caudal to the lesion site, using adeno-associated virus (AAV). Seven days after viral injection, contusions with 10 kD dextran pre-loading were performed rostral to the AAV-injected DRGs ( Fig. 7c ). One week later, normal appearing double-labelled axons (44±0.5% of all intact AAV-labelled axons; mean±s.e.m. ; n =105 axons, 3 mice) were found projecting through the thoracic spinal cord to the gracile nucleus, where these axons typically terminate ( Fig. 7d–f ). Here these recovered axons maintained varicosities, the vast majority of which were immune-positive for the presynaptic marker, vesicular glutamate transporters 1/2 ( Fig. 7d,e ). Taken together, these experiments indicate that a substantial fraction of axons that were disrupted by the initial impact and likely exposed to elevated calcium levels can reseal their plasma membrane, achieve calcium homeostasis and maintain their integrity and distal connectivity. Our in vivo fate analysis of individual axons after spinal cord contusion reveals that a substantial proportion of affected axons exist in a state of sublethal damage, from which they can either spontaneously recover or progress to degeneration. Importantly, this decision is open to intervention for at least a few hours after the impact. Such a neuropreservative intervention could be an important building block in a multistep therapeutic strategy, as axons that spontaneously recover from the initial insult maintain a long-distance connectivity and can thus provide a critical substrate for subsequent neurorestorative approaches. To understand how at-risk axons could be rescued after contusion, we studied whether calcium dyshomeostasis influences the fate of axons during the first hours after contusion. Concomitant in vivo monitoring of axonal calcium levels and morphology revealed that increases in axonal calcium levels precede fragmentation. Obviously, calcium per se is not a new or unexpected mediator of axonal demise, as previous studies have identified calcium as the proximate cause of subsequent axon degeneration in several disease and trauma models [2] , [12] . Our data for nontransecting trauma, however, support a more nuanced view, with calcium dysregulation and its resolution being a choice point of axonal fate. Indeed, we observed calcium rises in many axons early after spinal contusion; however, a substantial fraction of such axons managed to restore calcium homeostasis within 1 or 2 h. Axons that cleared calcium were almost completely protected from fragmentation. In contrast, axons with sustained calcium load fragmented at a high rate. Calcium-elevated axons after contusion thus appear to represent a metastable intermediate, which is capable of spontaneous resolution—rather than a precedent of imminent and immutable destruction. Given the critical role of calcium accumulations in contused axons, it is important to consider where the intra-axonal calcium is coming from and which downstream mechanisms it initiates. In vitro and in a multitude of neurological conditions, including trauma, ischaemia, inflammation and degeneration [12] , [26] , a broad range of mechanisms have been implicated as sources for elevated axonal calcium, including extracellular sources (for example, voltage-gated ion channels [17] , [18] , [19] , the plasma membrane sodium–calcium exchanger [20] , [21] , [22] , the acid sensing ion channel [27] or nodal glutamate receptors [23] ), as well as intracellular stores (such as mitochondria [28] or the endoplasmic reticulum [29] ). Our in vivo analysis now indicates that mechanoporation, that is, the formation of pores in the plasma membrane as first described after diffused brain injury [24] , is a dominant source of calcium influx at least in the first hours after contusion. On the basis of our dye-exclusion studies, such pores exist transiently, and the length of their persistence determines—together with the efficiency of calcium clearance—whether an axon degenerates or survives. Thus, interventions that seal pores might be beneficial after spinal contusion. However, a drug (polyethylene glycol) that has been suggested for such an intervention in other settings [25] did not improve resealing in our model ( Supplementary Fig. 3 ). Alternative intervention strategies could focus on either enhancing calcium clearance or blocking downstream destruction pathways, which likely provide a more easily targeted point of intervention than the pores themselves. Somewhat to our surprise we found that fragmentation in the immediate p.i period does not seem to be susceptible to the ‘Wallerian degeneration slow’ (WLD S ) fusion protein ( Supplementary Fig. 4 ), at least at the expression levels afforded by a highly axon-protective variant driven by a ubiquitous promotor (see Methods). Expression of this fusion protein blocks Wallerian degeneration and other forms of trauma-induced degeneration, as well as axon loss after nontransecting insults, such as ischaemia and toxin-induced neuropathy [2] , [30] , [31] . This suggests that pore-induced axon loss differs from the immediate (and WLD S -susceptible) acute axonal degeneration [16] observed after transection. Still, further downstream both mechanisms seem to converge on calcium-dependent proteases of the calpain family, as evidenced by block of axonal breakdown that we observed after calpain inhibitor application. Calpain inhibition per se is likely not a translatable therapeutic strategy (not least because calpain also mediates axonal membrane repair [32] ). However, our data directly demonstrate the existence of an at-risk axon population that can be rescued by applying calpain inhibitor during a limited period of time after injury (even though we do not know how many of these survive secondary injury cascades, such as delayed cell death, ischaemia or inflammation). Still these experiments make an important point: interventions might be efficacious in rescuing axons even if their application is delayed and their action transient—provided they are delivered at a time when a sufficient number of damaged axons in the indeterminate metastable state of calcium elevation still exists. Shifting the endogenous balance of recovery versus fragmentation in such an axonal population could rescue a noticeable fraction of them. As an interesting aside, the mechanopores induced by contusion could themselves act as entry ports for drugs, which in this way could be preferentially targeted towards at-risk axons (such drug-trapping might also explain the long-lasting protection against axonal fragmentation—for at least 8 h after injury—we observe after transient application of calpain inhibitor III). Our results demonstrate that a window of opportunity for neuropreservative interventions exists for several hours after contusion. The clinical potential of neuropreservative interventions is exemplified by the success of fibrinolysis therapy in stroke patients, which—if initiated within hours of vessel occlusion—can restore perfusion sufficiently to rescue neurons otherwise doomed to die [7] . Indeed, reversals of dendritic pathology have been observed by two-photon imaging after reperfusion in murine stroke models [33] . Just as stroke, a spinal trauma represents an easily recognizable acute medical emergency, and the initiation of an acute intervention in the first hours after injury thus appears feasible. While an intervention targeted at preserving axons through the acute post-traumatic period would not solve all problems of subsequent secondary changes, it should be noted that in our experiments a substantial fraction of initially damaged axons that survived the acute injury period persisted and maintained synaptic connectivity long term. Thus, promoting the rescue of at-risk axons early after spinal trauma might provide a first step of a multi-tiered therapeutic approach, which aims at preserving existing connectivity and providing an efficient substrate for subsequent replacement, regeneration or remodelling of axonal connections. Animals We used 2- to 6-month-old transgenic male and female mice to visualize axonal morphology ( Thy1 -YFP16; Jackson Laboratory strain Tg(Thy1-YFP)16Jrs/J ) [11] , [34] or to measure Ca 2+ dynamics ( Thy1 -TNXXL) [13] . Thy1 -TNXXL and ΔNLS R213AR215A WLD S (ref. 35 ) mice were maintained in a C57BL/6 background. C57BL/6 mice were used for tracing experiments. Thy1 -YFP16 mice were maintained on a mixed background. ΔNLS R213AR215A WLD S mice were crossed to Thy1 -TNXXL and F1 mice heterozygous for both transgenes were used for experimental analysis. The size distribution of axons of the Thy1 -YFP16 mouse line has been previously reported [34] . In the Thy1 -TNXXL mouse line, roughly half of the labelled axons on the dorsal surface have large diameters (>1 μm; Supplementary Fig. 1 ). Most of the thin axons in Thy1 -TNXXL mice are likely to be of intraspinal origin as they are rare in the dorsal roots. Animal experiments were conducted in accordance with local regulations and were approved by the responsible regulatory agencies. Surgical procedures Mice were anaesthetized by an intraperitoneal injection of ketamine–xylazine (ketamine 87 mg kg −1 , xylazine 13 mg kg −1 ). We performed spinal cord contusions using the Infinite Horizons Impactor (Precision Systems and Instrumentation) [10] . After a double dorsal laminectomy over the L4 and L5 segments, the mice were suspended using compact spinal cord clamps (Narishige) [36] . Contusion injuries were induced between the L4 and L5 vertebrae with a set force range from 30 to 35 kDynes (which resulted in an actual force range of 29–43 kDynes). Lesions with significant subdural bleeding that precluded microscopic observation, animals with weak lesions where no axons fragmented during the experimental time course or samples with significant movement artifact that could not be analysed were not used (44 of 105). In some samples, the lesion site was verified by spiking the artificial cerebrospinal fluid (aCSF) bath (2–3 ml) with 2 μl of a 0.56 mg ml −1 solution of ethidium homodimer-1 (Invitrogen) before or as much as 4 h after the lesion. In contusion experiments, vital dyes (1 μl of 3% TRITC-conjugated 10 kD dextran or 0.25–1 μl 2 mM AlexaFluor594-conjugated cadaverine for in vivo imaging, and 1 μl of 10% TRITC-conjugated 10 kD dextran or 10% TRITC-conjugated 3 kD dextran for survival experiments; all Invitrogen) were pressure-injected over 20–30 s subdurally using a hand-held pulled glass micropipette. To allow access of EGTA (25 mM in aCSF applied from 0 to 60 min), calpain inhibitor III (100 μM in aCSF from 60 to 120 min; Calbiochem), DMSO (0.5% in aCSF from 60 to 120 min or −30 to 60 min; Sigma-Aldrich), bepridil hydrochloride (200 μM in aCSF from −30 to 60 min; Sigma-Aldrich), nimodipine and ω-conotoxin GVIA (10 and 1 μM in aCSF from −30 to 60 min; Sigma-Aldrich and Tocris, respectively), CNQX disodium salt and MK 801 maleate (50 and 300 μM in aCSF from −30 to 60 min; Tocris) or polyethylene glycol (0.3 kD, 50% wt/wt in water from 0–5 min), small holes were made in the dura laterally at the rostral and/or caudal edges of the laminectomy using a dural hook fashioned from an insulin syringe. Images were always acquired contralateral to sites of dye injection or dural access. Pharmacological treatment was assigned before initiating surgical procedures. For backtracing of axons after spinal contusion, dorsolateral hemisections were performed at T8 using the tip of an insulin syringe. After axotomy, 1 μl of 10% fluorescein isothiocyanate (FITC)-conjugated 3 kD dextran was loaded into the lesion site by pressure injection through a pulled glass micropipette over 30–60 s. For AAV injections into DRGs, mice were anaesthetized with 0.05 mg kg −1 fentanyl, 5 mg kg −1 midazolam and 0.5 mg kg −1 medetomidin, and the left or right L5 or L6 DRG was exposed by dorsal laminectomy. Half a microlitre of an AAV-CAG-cyan fluorescent protein (CFP) virus (see below; titre: 8 × 10 12 genome copies per ml, diluted 1:5 in sterile PBS) was slowly injected into the DRG through a pulled glass micropipette. Virus production The coding sequence for CFP was cloned into the pAAV-CAG-MCS vector from Stratagene. AVV was produced by the adenovirus-free AAV production method as previously described [37] . Histology and immunohistochemistry After transcardiac perfusion of mice with 4% (wt/vol) paraformaldehyde in PBS, spinal cords were post-fixed for 12–24 h. Spinal cords, brainstems and DRGs were dissected. The lesion site and DRGs were imaged as whole mounts, while spinal cords and brainstems were sectioned on a vibratome. Immunofluorescence stainings for CFP, and vesicular glutamate transporter 1/2 (Vglut1/2), were performed at room temperature using free-floating tissue sections. After three washes in PBS, sections were blocked and permeabilized in blocking solution (5% normal goat serum, 5% bovine serum albumin and 0.2% Triton X-100 in PBS) for 1 h. Primary antibodies (chicken anti-GFP (green fluorescent protein), Chemicon A10262, 1:1,000; rabbit anti-Vglut1/2, Synaptic Systems 135-503, 1:400) were incubated overnight in blocking solution. After three washes with PBS, we incubated the sections in blocking solution containing secondary antibody (AlexaFluor488-conjugated goat anti-chicken; AlexaFluor647-conjugated goat anti-rabbit; 1:1,000; Invitrogen) for 1 h. Sections were mounted in mounting medium (Vectashield) before confocal imaging. In vivo imaging and analysis In vivo imaging of the lumbar spinal cord was carried out as previously described [34] , [38] . Briefly, mice were anaesthetized by an intraperitoneal injection of ketamine–xylazine (ketamine 87 mg kg −1 , xylazine 13 mg kg −1 ). Anaesthesia was reapplied as needed (60–120 min). To access the dorsal surface of the lumbar spinal cord, a laminectomy was performed. To minimize movement during high-resolution imaging, the vertebral column was immobilized using compact spinal cord clamps (Narishige) [36] . Symmetrical incisions were made lateral to the spinal column, one pair along the vertebral level rostral, and another pair two segments caudal to the laminectomy site for insertion of the spinal cord clamps. To allow for the formation of a liquid reservoir (regularly filled with pre-warmed mouse aCSF: 148.2 NaCl, 3.0 KCl, 1.4 CaCl 2 , 0.8 MgCl 2 , 0.8 Na 2 HPO 4 and 0.2 NaH 2 PO 4 in mM) and access with a water-dipping-cone microscope objective (× 25/1.05), an agarose well (2% agarose in aCSF) was made around the surgery site. Image stacks were acquired using a commercially available Olympus FV1000 MPE equipped with a femto-second pulsed Ti:Sapphire Laser (Mai Tai HP, Newport/Spectra-Physics). The laser was tuned to 920 nm for excitation of YFP or 840 nm for measurement of calcium dynamics and for vital dye observations. Detectors consisted of either conventional or gallium arsenide phosphide (GaAsP) photomultiplier tubes. All light was first filtered through a 690-nm short pass dichroic mirror. A 540/40-nm barrier filter in front of the GaAsP detectors was used for imaging YFP. For imaging FRET signals in Thy1 -TNXXL mice, we used a CFP/YFP cube consisting of a 505-nm dichroic mirror to separate CFP and cpCitrine signals and 480/40- and 540/40-nm filter sets in front of the photomultiplier tubes. For imaging FRET signals and vital dyes, emission light was first passed through a 565-nm short pass dichroic mirror, the CFP/YFP cube was positioned in front of GaAsP detectors and a 602.5/55-nm barrier filter was positioned in front of a conventional photomultiplier tubes to detect red signals. Immediately after spinal contusion, mice were transported from the impactor device to the microscope. The first images after contusion were then acquired between 2 and 8 min after lesion. To aid in finding back the same region as mice were removed from the set-up, an autofluorescence image was acquired using a very low power 405 nm laser for sample excitation and light collection along the multiphoton light path. This creates a negative vascular image, which allows re-aligning the sample. Image stacks were acquired as pairs with roughly 10–20 μm of overlap along the rostrocaudal axis at 10 min intervals at a pixel size of 397 nm, and a 0.7- to 0.8-μm z-step yielding a total volume of roughly 500 × 250 × 50 μm. Experiments were carried out for 4 h (in selected cases for up to 8 h). We have previously demonstrated that phototoxicity does not appear to have an impact on the health of spinal axons under such imaging conditions [34] , [38] . Images were post-processed using the open-source image analysis software, Fiji [39] , and the image-processing software, Photoshop (Adobe). Each image stack was z-projected using a maximum intensity projection, visualized using a black-grey look-up table for Thy1 -YFP16 or pseudocolours for the CFP and cpCitrine channels for Thy1 -TNXXL, and the look-up table adjusted accordingly along a linear scale. Resultant images were manually stitched together as two-panel montages in Photoshop. These montages where then built into a temporal image stack in Fiji and registered using the ‘SIFT’ plug-in in Fiji constrained to XY-translation. Morphological state and calcium measurements were recorded for any axon that could be tracked along the entire time course. In treatment experiments the observer was blinded to the treatment status of the animal. For an axon to be included in the analysis it must have been observable across all time points during the 4-h time-lapse over at least 50 μm. It should be noted that this selection criterion may bias the analysis towards brighter axons, and those that do not fragment. Collateral neurites running laterally across the spinal cord were not included in our analysis because in most cases they degenerated immediately after contusion, and in many instances could be traced to a cell soma indicating that they may be dendrites. This makes up only a small population of neurites on the dorsal surface (one to two per sample). Following analysis in z-projections, each transition was verified by observations of morphology and measurements of FRET signals within unprocessed three-dimensional (3D) image stacks. In Thy1 -TNXXL mice, FRET measurements of all tracked axons were made before injury, at the first time point after contusion, at the final time point of the time-lapse and at any pair of time points when a transition was recorded. Local background-subtracted FRET measurements were made at the location where the cpCitrine/CFP ratio appeared to be the highest, and axons were considered to be Ca 2+ -elevated if ratios were locally elevated or if they were elevated across the entire observable length of the axon. An axon was scored as having elevated Ca 2+ levels if the cpCitrine/CFP ratio was 50% greater than its pre-injury ratio. If a FRET measurement revealed a transition scored by visual inspection to be incorrect, measurements were made across time points until the moment of transition was accurately placed. We chose this binary scoring approach because the relatively steep sigmoidal response curve of genetically encoded calcium indicators and their relatively low K d compared with extracellular calcium concentrations precludes an informative measurement of the actual calcium levels inside injured axons in our setting. We verified that the FRET ratios were not influenced by pH changes after injury by performing injuries in Thy1 -YFP16 × Thy1 -CFP5 mice (where YFP acts as a pH sensor). Fluorescence ratios measured in these mice were not altered 2 h after contusion (post/pre=0.99±0.02, three mice, 99 axons). Axonal fragmentation was also verified by examining 3D image stacks that were optimally contrast-adjusted for the axon in question, alongside two-dimenstional time-lapse data. This two-part approach is important because ‘pulling apart’ behaviour seen in the time-lapse can indicate that an axon is fragmenting. However, in some cases fine processes indicating axonal continuity are not apparent in z-projections, and are only observable in contrast-adjusted image stacks. We have addressed the veracity of axonal fragmentation apparent from in vivo fluorescent microscopic observations in our previous papers [16] , [34] , [40] . The main arguments for our interpretation that clearly identifiable gaps in fluorescence contiguity correspond to actual axon discontinuities are: (1) in chronic experiments, where such gaps were identified by us [16] and others [41] , subsequent Wallerian degeneration of the axon segment distal to the gap in fluorescence was observed. (2) If combined with functional sensors, injuries that cause gaps in fluorescence generally correspond with signals expected to arise from plasma membrane disruptions (for example, ion influx, mitochondrial damage and so on) that spread in a predictable pattern away from the gap [42] . Indeed, even with purely morphological labelling, one important factor in scoring a broken axon is a ‘pulling apart’ movement of either side of the putative fragmentation point. (3) In studies correlating in vivo with post hoc confocal or electron microscopy 3D reconstructions, gaps in continuity seen in vivo could generally be confirmed by higher contrast and resolution methods [16] , [34] , [40] . The rare instances where ambiguities remain were excluded from analysis. Experiments with pharmacological manipulations were scored by a blinded observer except for EGTA, which was obvious, given the large suppression of calcium elevations in these samples. Five Thy1 -TNXXL mice (177 axons) were examined by independent scorers in order to assess inter-rater reliability. The following disparity rates were observed (as percentage of all axons in this category): swelling 2.8±2.0%; elevation 5.1±1.6%; recovery 4.0±1.9%; breakdown 6.2±2.7%; and return 2.1±1.5% (mean±s.e.m.). To assess the uptake of vital dyes, axonal intensity measurements of 30% or more above the local background were scored as dye-positive. Confocal microscopy and analysis We obtained confocal images of fixed samples on an FV1000 confocal scan-head mounted on an upright BX61 microscope (Olympus). To create overviews of the lesion site, a block of fixed tissue four to five spinal segments in length was secured with its dorsal surface to a cover glass in 2% agarose. This ‘hanging-drop’ preparation was scanned with a × 4/0.13 air objective at 3.105-μm pixel size. Higher power and full-resolution images using oil objectives of regions that had been imaged in vivo were also acquired in these preparations. For retrograde tracing experiments, the two DRGs, the axons of which entered via the dorsal root directly caudal to the lesion were analysed, along with the DRGs three segments rostral to the lesion, which were used as normalization for back-tracing efficiency. Only DRGs contralateral to the contusion dye (TRITC)-loading side were used to prevent labelling caused by the dye injection. DRGs were scanned as whole mounts in Vectashield using a × 10/0.4 air objective at 530-nm pixel size and 2-μm spacing of z-sections. Line serial acquisition was used to prevent spectral bleed-through of FITC and TRITC probes. Raw stacks were analysed by hand by blinded observers in Fiji using the cell counter plug-in. The volume of each DRG was measured by taking an area measurement of the DRG boundaries of each optical section and multiplying by the z-section spacing. For estimates of axon loss by contusion, the density of FITC labelling was measured in the rostral DRG, and the densities in each caudal block were divided by the rostral density to normalize for back-tracing efficiency (10 DRGs, five mice). These measurements were compared with samples from sham-operated non-contused mice (10 DRGs, five mice). Contusion led to a 47±7% (mean±s.e.m. ; n =5 mice per group) reduction in back-tracing efficiency relative to sham-operated mice. To assay the long-term maintenance of axon projections, the brainstems, spinal cords and DRGs of animals were examined. The extent of CFP expression within the targeted DRG was verified by whole-mount imaging as above. The entry point of axons through the dorsal root caudal to the lesion site was verified using the agarose hanging-drop preparation as described above. Axons passing through the thoracic spinal cord were scanned in 50-μm-thick vibratome sections with a × 60/1.42 oil immersion objective at a pixel size of 132 nm and a z-section spacing of 400 or 500 nm. CFP and TRITC signals were scanned using ‘line sequential’ scanning to avoid spectral bleed-through. Sections were imaged serially anchored on the caudal edge of the section to avoid double counting of axons. The ‘Cell Counter’ tool in Fiji was used to manually count axons positive for AAV or both AAV and TRITC in unenhanced samples. Forty-micrometre-thick coronal sections of the brainstem that had been immunostained for GFP to enhance native signal and VGlut1/2 to identify synaptic terminals were scanned with a × 60/1.42 oil immersion objective at a pixel size of 207 nm and a z-section spacing of 500 nm. Raw images were analysed manually with the ‘Cell Counter’ tool in Fiji by first tagging boutons identified on the basis of the CFP signal, and then determining which of these boutons were also TRITC-positive. With only the CFP tags displayed, the presence or absence of Vglut1/2 signal was scored. Some images were rotated in 3D visualization software (Amira) or were median-filtered for clearer display purposes in figure panels. For display consistency, some images were reflected such that the dorsal roots were consistently towards the bottom of figure panels. All text overlaying images is superimposed on a semitransparent dark box, the borders of which were obscured with Gaussian blur in order to improve legibility while preserving data beneath text. Statistical analyses Results are given as mean±s.e.m. Statistical significance was determined with the GraphPad Prism 5 software using bilateral Mann–Whitney tests as normal distributions could not be confirmed. Sample sizes were chosen on the basis of previous experience using similar methodologies [34] . How to cite this article: Williams, P. R. et al . A recoverable state of axon injury persists for hours after spinal cord contusion in vivo . Nat. Commun. 5:5683 doi: 10.1038/ncomms6683 (2014).